Advection shapes Southern Ocean microbial assemblages independent of distance and environment effects Although environmental selection and spatial separation have been shown to shape the distribution and abundance of marine microorganisms, the effects of advection (physical transport) have not been directly tested. Here we examine 25 samples covering all major water masses of the Southern Ocean to determine the effects of advection on microbial biogeography. Even when environmental factors and spatial separation are controlled for, there is a positive correlation between advection distance and taxonomic dissimilarity, indicating that an ‘advection effect’ has a role in shaping marine microbial community composition. This effect is likely due to the advection of cells increasing the probability that upstream microorganisms will colonize downstream sites. Our study shows that in addition to distance and environmental selection, advection shapes the composition of marine microbial communities. The central goal of microbial biogeography is to understand how the distribution and abundance of microorganisms are shaped by their physical context. The Baas Becking hypothesis—that ‘ everything is everywhere , but, the environment selects [1] , [2] ,—posits that the rapid dispersal of microorganisms means microbial community structure is determined entirely by environmental selection. This stands in contrast to macroorganism biogeography, which has long been recognized as being under the control of historical (in addition to contemporary environmental) factors, particularly spatial influences such as barriers to dispersal. Microbial biogeography studies have begun to show that historical factors may also shape the distribution of microorganisms [3] , for example, a correlation between spatial and genetic distance (a ‘distance effect’) in fluorescent Pseudomonas strains in soils [4] . This study, among others [5] , [6] , also demonstrated the importance of taxonomic resolution in describing such biogeographic patterns. Other studies have found that dispersal potential varies between microbial species, leading to different or absent distance effects [7] . When combined with contemporary environmental selection (‘environment effect’), distance effects explain some but not all variation between microbial communities, and the mechanism(s) by which a distance effect arises are not always clear [8] . In the ocean, several recent studies have found that microbial communities can be endemic to hydrographically distinct water masses. Surveys in the Arctic [9] and North Atlantic [10] oceans have found that bacterial assemblages within the same water mass can be similar across a range of thousands of kilometres, but assemblages can differ between water masses across a range of hundreds of metres. Water masses are defined by their distinct physicochemical properties; hence, such patterns do not directly imply the existence of factors beyond environmental selection. However, in some cases a water mass–community relationship has been shown to persist even when environment effects are statistically controlled for [11] , [12] . One explanation for these results is that microbial assemblages are influenced by the advection (physical transport) of cells by ocean currents. Higher dispersal rates cause the microbial community composition at a given site to increasingly resemble the dispersed colonizers, and less reflect local environmental selection and stochastic effects such as genetic drift [8] . Hence, it would be expected that locations that are closely connected by advection would have more similar compositions than those that are not, even when the environment effect is accounted for. Indeed, advection is often invoked to explain observations of microbial diversity or abundance, which do not seem attributable to environmental selection (for example, refs 13 , 14 , 15 , 16 ). The exchange of very small volumes of water between marine microbial mesocosms has been found to greatly reduce their β-diversity (in this case, compositional differences between communities from different mesocosms) even under consistent environmental conditions [17] . This suggests that advection of even small numbers of cells could have a large homogenizing effect independent of environmental selection. However, the existence of a relationship between advection and community composition that is independent of environment and distance effects has not been directly tested. The Southern Ocean (SO) is composed of several water masses, which are physicochemically distinct but linked by circulation [18] ( Fig. 1 ). Oxygen-depleted Upper Circumpolar Deep Water (CDW), originating in the deep Indian and Pacific oceans [19] , and high-salinity Lower CDW originating in the Atlantic, spread polewards and shoal to reach the sea surface of Antarctic Zone (AZ) waters between the Polar Front and the Antarctic continent. Some of the upwelled CDW moves southwards, where it becomes colder and denser and sinks to form Antarctic Bottom Water (AABW), which spreads northwards to ventilate the densest layers of the global ocean. The remainder of the upwelled water is warmed and freshened as it moves northwards before sinking to form Antarctic Intermediate Water (AAIW), which spreads northwards at about 1,000 m depth. Overlying the AAIW is the warmer Subantarctic Mode Water (SAMW). 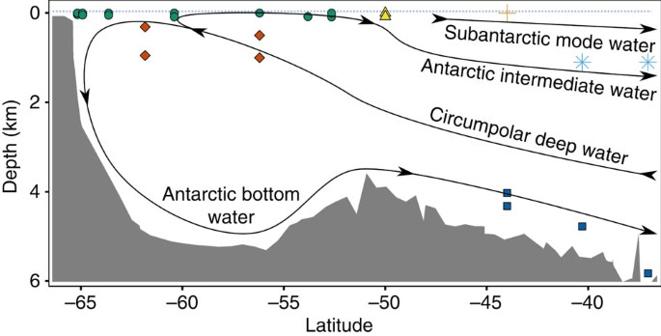Figure 1: Map of SO sample locations. AAIW, light blue stars; SAMW, orange crosses; AABW, dark blue squares; AZ, green circles; PFZ, yellow triangles; CDW, red diamonds; sea surface, blue dashed horizontal line. Bathymetry is an approximate representation for 115° E, and is indicative only. Figure 1: Map of SO sample locations. AAIW, light blue stars; SAMW, orange crosses; AABW, dark blue squares; AZ, green circles; PFZ, yellow triangles; CDW, red diamonds; sea surface, blue dashed horizontal line. Bathymetry is an approximate representation for 115° E, and is indicative only. Full size image This study aims to determine whether advection shapes the community structure of bacteria and archaea, independent of environment and distance effects. By sampling each of the SO water masses (depths from surface to ≈6 km), we compare microbial communities over a large spatial distance (≈3,000 km) and range of environments, and test whether advection has a role in shaping their composition. When environment and distance effects are controlled for, a significant correlation between advection distance and community dissimilarity is observed. The findings indicate that advection shapes marine microbial community composition. Sequencing and taxonomic assignment After trimming, denoising and chimera removal, the 25 samples (each with three separately sequenced size fractions) yielded 1,008,963 16S ribosomal RNA gene pyrosequencing reads of length 251–561 bp (mean 426 bp). Individual fractions yielded 3,687–52,192 reads (mean 13,453). After preprocessing in Quantitative Insights Into Microbial Ecology (QIIME), 2,473–45,046 (mean 11,599) reads per fraction were retained. Operational taxonomic units (OTUs) were identified by clustering reads at a minimum sequence identity of 97%, broadly equivalent to the species level. This threshold has been widely used for the delineation of bacterial species, allowing our results to be compared with past and future studies that adopt this criterion. Unique OTUs (15,868) were identified across all fractions of all samples, 13,011 of which were generated de novo ; that is, they did not cluster with sequences in the SILVA database. In many samples and size fractions, the total abundance of OTUs generated de novo was greater than that of OTUs identified by clustering with SILVA seed sequences ( Fig. 2 ). However, the mean relative abundance of individual OTUs that clustered with SILVA was higher (2.1%) than that of OTUs generated de novo (0.43%). This suggests that although there exists a ‘long tail’ of many rare OTUs that are not in SILVA, the most abundant OTUs in the sampled environments are well represented in SILVA. The Chao 1 statistic was calculated, and estimated OTUs were undersequenced by 1.5–51% across all samples (mean 37%; Supplementary Data 1 ). 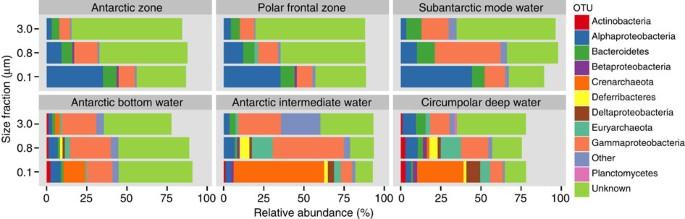Figure 2: Taxonomic assignments for each sampled water mass. Relative abundances of OTUs in each sampled water mass and size fraction. OTUs that formed by clustering against SILVA 16S rRNA gene seed sequences were aggregated to the phyla associated with those sequences, except for members of the Proteobacteria, which were aggregated to class when known. OTUs generated byde novoclustering were aggregated as ‘unknown’. For ease of comprehension, phyla or classes with a mean relative abundance across all samples and fractions <1% were aggregated into a single group labelled ‘other’. Relative abundance was scaled to account for discarded reads. Surface water masses are in the top row and deeper water masses are in the bottom row. Figure 2: Taxonomic assignments for each sampled water mass. Relative abundances of OTUs in each sampled water mass and size fraction. OTUs that formed by clustering against SILVA 16S rRNA gene seed sequences were aggregated to the phyla associated with those sequences, except for members of the Proteobacteria, which were aggregated to class when known. OTUs generated by de novo clustering were aggregated as ‘unknown’. For ease of comprehension, phyla or classes with a mean relative abundance across all samples and fractions <1% were aggregated into a single group labelled ‘other’. Relative abundance was scaled to account for discarded reads. Surface water masses are in the top row and deeper water masses are in the bottom row. Full size image Non-metric multidimensional scaling (nMDS) ordination showed that the sampled water masses could be distinguished on the basis of taxonomic distance ( Fig. 3c ). This was supported by the analysis of similarity (ANOSIM; R =0.83, P =0.001). Although each water mass had a distinct taxonomic profile, some broad differences between surface and deep masses were observed ( Fig. 2 ). Surface waters (AZ, Polar Frontal Zone (PFZ) and SAMW) had high abundances of OTUs clustering with SILVA sequences from the Alphaproteobacteria, Bacteroidetes and Gammaproteobacteria. The higher abundance of Bacteroidetes at the surface reflects their association with phytoplankton, as many species in this lineage specialize in the degradation of high molecular weight products of primary production [20] . Alphaproteobacteria were represented primarily by the SAR11 clade, abundant in ocean surface communities [21] including the SO [22] , and Roseobacter clades, which have also been associated with degradation of phytoplankton products [15] , [20] ( Supplementary Data 2 ). The dominant Gammaproteobacterial orders were the Alteromonadales and Oceanospirillales, typical of SO surface waters [23] . Archaeal OTUs were not abundant at the surface, consistent with their well-described decline in abundance during summer [24] , [25] . The deep water masses (CDW, AAIW and AABW) were dominated by Crenarchaeota, Euryarchaeota and Gammaproteobacteria, again consistent with previous findings [26] . 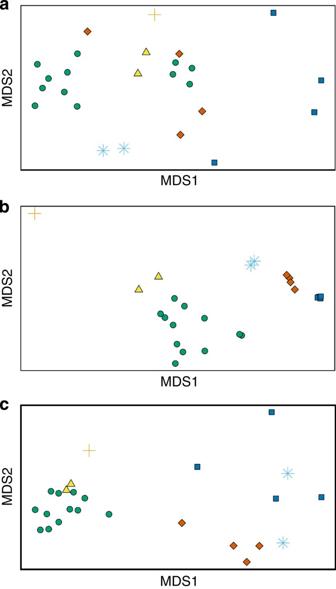Figure 3: nMDS ordinations. First two nMDS dimensions of the (a) advection (2D stress=0.19), (b) environmental (2D stress=0.02) and (c) taxonomic (2D stress=0.08) distance/dissimilarity matrices. AAIW, light blue stars; SAMW, orange crosses; AABW, dark blue squares; AZ, green circles; PFZ, yellow triangles; CDW, red diamonds. Figure 3: nMDS ordinations. First two nMDS dimensions of the ( a ) advection (2D stress=0.19), ( b ) environmental (2D stress=0.02) and ( c ) taxonomic (2D stress=0.08) distance/dissimilarity matrices. AAIW, light blue stars; SAMW, orange crosses; AABW, dark blue squares; AZ, green circles; PFZ, yellow triangles; CDW, red diamonds. Full size image Environment and distance effects nMDS ordination showed that the sampled water masses clustered well on the basis of environmental distance ( Fig. 3b ). This was supported by ANOSIM ( R =0.84, P =0.001). A partial Mantel test, comparing the taxonomic to environmental matrices with the spatial matrix held constant, found a correlation of r =0.54 ( P =0.001), indicating a strong environment effect. Distance-based linear models (distLM) analysis of the individual physicochemical variables found that considered separately, each of phosphate, silicate, nitrate, oxygen, salinity and pressure explained 12–25% of the taxonomic variance between samples ( P =0.001–0.002). Temperature had no significant effect on taxonomic composition when considered separately ( P >0.05). When all combinations of variables were considered (BEST modelling), the full set of variables was found to be a better solution (adjusted R 2 =0.33) than any subset. This suggests that no redundant physicochemical parameters were measured. The distance-based redundancy analysis (dbRDA) plot showed that the physicochemical parameters structured the samples first along an axis separating surface and deep samples (dbRDA1), strongly related to dissolved oxygen ( r =0.72; Fig. 4 ). The second axis was best correlated with temperature ( r =0.91). All variables had a moderate correlation with at least one of the first two axes ( Supplementary Data 3 ). As with the nMDS ordinations ( Fig. 3 ), the water masses were generally well separated by the first two dbRDA axes. Samples from the AABW and AAIW, which were not well separated by the first two axes, were clearly separated along the third ( Supplementary Data 3 ), which was best correlated with silicate ( r =−0.77), reflecting the relative enrichment of silicate in the AABW. 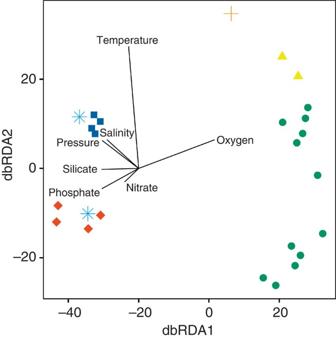Figure 4: Relationship between physicochemical variables and sample taxonomic composition. dbRDA ordination of the distLM model describing the relationship between physicochemical variables and the taxonomic dissimilarity between samples. Vectors represent the effect of each predictor variable on the two visualized axes. Vector length corresponds to the relative size of the effect, whereas direction represents the correlations to the two displayed axes. The first axis (dbRDA1) captures 51% of fitted and 26% of total variation between the samples’ taxonomic profiles; the second (dbRDA2) captures 16% of fitted and 8% of total variation. AAIW, light blue stars; SAMW, orange crosses; AABW, dark blue squares; AZ, green circles; PFZ, yellow triangles; CDW, red diamonds. Figure 4: Relationship between physicochemical variables and sample taxonomic composition. dbRDA ordination of the distLM model describing the relationship between physicochemical variables and the taxonomic dissimilarity between samples. Vectors represent the effect of each predictor variable on the two visualized axes. Vector length corresponds to the relative size of the effect, whereas direction represents the correlations to the two displayed axes. The first axis (dbRDA1) captures 51% of fitted and 26% of total variation between the samples’ taxonomic profiles; the second (dbRDA2) captures 16% of fitted and 8% of total variation. AAIW, light blue stars; SAMW, orange crosses; AABW, dark blue squares; AZ, green circles; PFZ, yellow triangles; CDW, red diamonds. Full size image A distance effect was detected by comparing the taxonomic and spatial matrices with the environmental matrix held constant (partial Mantel; r =0.41, P =0.003). This indicated that a process other than contemporary environmental selection was appreciably affecting variation in the microbial community composition. Testing of advection effect Encounters (244,000) were recorded between particles and sample sites during the 100-year advection simulation. Encounter times spanned the full range of the simulation (5 days–100 years), with a median of 30 days and mean of 3,018 days. Forty-seven pairs of samples did not yield mutual encounters (that is, at least one particle from one sample encountering the other). Of these, every pair included at least one AABW sample. nMDS ordination showed that the sampled water masses could be broadly distinguished on the basis of their mutual advection distances ( Fig. 3a ). This was supported by ANOSIM ( R =0.41, P =0.002). A partial Mantel test, comparing the taxonomic and advection matrices with the spatial and environmental matrices held constant, showed that advection has a moderate ( r =0.28) and significant ( P =0.01) correlation with taxonomic composition independent of spatial and environmental factors. To ensure this result was not unduly influenced by the samples on which the 100-year ceiling was imposed (AABW), and those for which particle releases were not simulated (samples 11, 13, 17 and 22), the test was repeated with these samples removed. The correlation was stronger and remained significant ( r =0.34, P =0.03). To ensure that the result was robust to the choice of advection distance metric, correlations were recalculated for both the full set of samples and the subset (excluding AABW and samples 11, 13, 17 and 22) with pairwise advection distance redefined as the mean time for all particle encounters between samples. The observed correlation was higher using this metric for both the full set ( r =0.41, P =0.004) and subset ( r =0.50, P =0.005). Source Tracker analysis confirmed that the effect was moderately directional, with the proportion of OTUs contributed from a given ‘source’ sample to a ‘sink’ sample correlated with the proportion of particle encounters it generated (Spearman’s ρ =0.15, P =0.001). To explore the role of taxonomic resolution in the detection of an advection effect, partial Mantel tests were repeated as above with OTUs clustered at different sequence similarity thresholds (0.80, 0.85, 0.90, 0.95, 0.99 and 1.00). The advection effect (as measured by the magnitude of the partial Mantel correlation) was strongest at a sequence similarity threshold of 0.90 ( r =0.31, P =0.01), decreasing in both directions from this maximum ( Fig. 5 ). 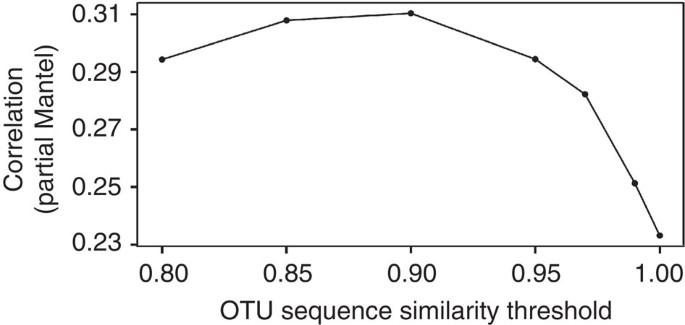Figure 5: Taxonomic resolution. Effect of taxonomic resolution (OTU clustering sequence similarity threshold) on partial Mantel correlation (r) between advection and taxonomic distances, with environmental and spatial distances held constant. All correlations are statistically significant (right-tailedPfrom 999 permutations <0.05). The full set of 25 samples was used. Figure 5: Taxonomic resolution. Effect of taxonomic resolution (OTU clustering sequence similarity threshold) on partial Mantel correlation ( r ) between advection and taxonomic distances, with environmental and spatial distances held constant. All correlations are statistically significant (right-tailed P from 999 permutations <0.05). The full set of 25 samples was used. Full size image Explaining the advection effect Two explanations can be proposed for the relationship between advection and community composition. The first is that advection increases microbial dispersal by increasing the probability that OTUs from one site will encounter and colonize another (the ‘dispersal mechanism’). This assumes microbial dispersal is less than perfect; that is, ‘everything is not everywhere’. The second possibility is that advection transports a large numbers of cells at a rate measurably outpacing environmental selection, regardless of whether or not those cells are able to successfully colonize (that is, grow and reproduce in) downstream sites: that ‘the environment selects, but not fast enough’ (the ‘bulk transport mechanism’). Considering the long advection times between sites in this study, the relatively rapid growth of marine microorganisms and the ability of small numbers of cells to rapidly reduce β-diversity between isolated marine sites [17] , the dispersal mechanism seems to be more plausible. Two tests were performed to distinguish between these hypotheses. First, the advection distance matrix was reconstructed using the absolute pairwise number of particle encounters as the distance metric between samples (distance metric for given sample pair=maximum number of encounters across all sample pairs−encounters for given pair+1). There was no significant correlation between this matrix and the taxonomic distance matrix when the environmental and spatial matrices were held constant ( P >0.05). This suggests that advection time, not the absolute number of transported cells, is the relevant factor, supporting the dispersal mechanism. Second, it was reasoned that under the dispersal mechanism, advection would have a large effect on the presence and diversity of taxa and a smaller effect on their abundances, whereas if the bulk transport hypothesis held, the effect would largely be on the relative abundances. To test this, the taxonomic profiles were transformed to a presence/absence measure (OTU present=1, absent=0), and a matrix of Sørensen dissimilarities were generated. The advection effect was slightly stronger ( r =0.29, P =0.009) than when abundances were considered, again supporting the dispersal hypothesis. The hypothesis that advection shapes microbial assemblages independent of an environment or distance effect is supported by our analyses of SO communities ( Figs 1 , 2 , 3 , 4 , 5 ). Communities that are more closely connected by advection are more similar, and this effect exists even when environment and distance effects are controlled for. Our analyses also indicate that advection primarily shapes microbial community structure by increasing opportunities for colonization, rather than transporting large numbers of cells to downstream sites. The amount of variance in taxonomic composition explained by the advection effect can be estimated as the square of the correlation coefficient ( r 2 ). This value, 8%, is likely to be a conservative estimate, as our study only captured advective pathways from one sample to another; it is possible that some samples with a large mutual advective distance shared a common advective source outside the study area. A recent review of studies partitioning variance in microbial community composition found that the mean reported variance explained by a distance effect was 10% and by an environment effect 27% (ref. 8 ). The estimated proportions of variance in our study, 17% ( P =0.003) for distance and 29% ( P =0.001) for environment, were close to these values, with the larger than average distance effect likely because of the large spatial scale of this study. Although there are no comparative data for the advection effect in other systems, the value of at least 8% for the SO indicates that advection is important relative to both distance and environment effects. Taxonomic resolution (that is, the level of genetic difference at which OTUs are discriminated) often determines whether or not a pattern is detected in studies of microbial distance effects, with finer resolutions generally leading to an increased likelihood of detecting a significant effect [8] . Although this held true in this study for OTU clustering thresholds of 0.80–0.90, OTU profiles generated with thresholds finer than 0.90 had decreasing correlations to advection, although they remained statistically significant ( Fig. 5 ). There are several factors that may contribute to this pattern. At very fine (0.99 and 1.00) clustering thresholds, sequencing error may increase random noise within the OTU profiles. As the V6–V8 hypervariable regions were selected as the sequencing target, it may also be attributed to intraspecific variation in 16S rRNA gene sequences within established populations [27] , which could increase the apparent divergence between sampled communities. Although such variation is unlikely to accumulate during the relatively short advection times observed in this study (median encounter time 30 days), it is consistent with advection as a historical factor increasing the chance of colonizers from ‘upstream’ sites reaching and establishing long-term populations in ‘downstream’ sites. However, as it is unlikely that intraspecific variation would have an effect at thresholds<0.97, this pattern of decreasing effect at taxonomic resolutions finer than 0.90 should be further investigated. To obtain a better understanding of the advection effect, it would be useful to determine whether specific taxonomic or physiological groups are more amenable to dispersal by advection; for example, through the formation of dormant spores [7] , [13] , copiotroph resting states (for example, Photobacterium angustum [28] ) or through the inherent stress resistance states of some oligotrophs (for example, Sphingopyxis alaskensis [28] ). As it is possible that an unmeasured environmental variable (for example, iron concentration; microenvironmental factors owing to particle attachment) also correlates with both advection and community composition, future studies should address this. Mesocosm experiments [17] may also help to address the effects of small-scale exchanges of cells on community structure. Although future work will help to clarify the nature of the advection effect, our data indicate that advection should be considered alongside distance and environment effects in studies addressing factors that shape marine microbial assemblages. Sampling Sampling was conducted on board the RSV Aurora Australis during cruise V3 from 20 January to 7 February 2012. This cruise occupied a latitudinal transect from waters north of Cape Poinsett, Antarctica (65° S) to south of Cape Leeuwin, Australia (37° S) within a longitudinal range of 113–115° E. Sampling was performed as described in ref. 29 , with sites and depths selected to provide coverage of all major SO water masses. At each surface station, ≈250–560 l of seawater was pumped from ≈1.5 to 2.5 m depth. At some surface stations, an additional sample was taken from the Deep Chlorophyll Maximum (DCM), as determined by chlorophyll fluorescence measurements taken from a conductivity, temperature and depth probe (CTD) cast at each sampling station. Samples of mesopelagic and deeper waters (≈120–240 l) were also collected at some stations using Niskin bottles attached to the CTD. Sampling depths were selected based on temperature, salinity and dissolved oxygen profiles to capture water from the targeted water masses. Profiles were generated on the CTD descent, and samples were collected on the ascent at the selected depths. Deep water masses were identified by the following criteria: CDW=oxygen minimum (Upper Circumpolar Deep) or salinity maximum (Lower Circumpolar Deep); AABW=deep potential temperature minimum; AAIW=salinity minimum [18] . The major fronts of the SO, which coincide with strong horizontal gradients in temperature and salinity [19] , [30] , separate regions with similar surface water properties. The AZ lies south of the Polar Front (which was at 51° S during sampling), whereas the PFZ lies between the Polar Front and the Subantarctic Front. In total, 25 samples from the AZ, PFZ, SAMW, AAIW, CDW and AABW were collected for this study ( Fig. 1 , Supplementary Data 1 ). Seawater samples were prefiltered through a 20-μm plankton net, biomass captured on sequential 3.0-, 0.8- and 0.1-μm 293-mm polyethersulphone membrane filters and filters immediately stored at −80 °C [31] , [32] . DNA extraction and sequencing DNA was extracted with a modified version of the phenol-chloroform method [31] . Tag pyrosequencing was performed by Research and Testing Laboratory (Lubbock, USA) on a GS FLX+ platform (Roche, Branford, USA) using a modification of the standard 926F/1392R primers targeting the V6–V8 hypervariable regions of bacterial and archaeal 16S rRNA genes (926wF: 5′-AAA-CTY-AAA-KGA-ATT-GRC-GG-3′, 1,392 R: 5′-ACG-GGC-GGT-GTG-TRC-3′). Denoising, chimera removal and trimming of poor quality read ends were performed by the sequencing facility. Generation of taxonomic dissimilarity matrix Using QIIME 1.6.0 (ref. 33 ), tag pyrosequencing reads were clustered into OTUs with >97% sequence similarity using the uclust_ref algorithm [34] , with rRNA gene sequences from the SILVA database (release 108, eukaryote and chloroplast sequences removed) [35] used as seed sequences and de novo cluster formation (that is, formation of clusters with no seed sequence) allowed. Following the QIIME default settings, reads with mean quality scores <25, homopolymer runs >6 nucleotides in length or errors in the primer sequence were discarded during preprocessing. To generate a taxonomic profile for each sample, the relative abundances of reads assigned to each OTU in each size fraction were encoded as variables. To account for the reads discarded by QIIME, abundances in each size fraction were standardized by the proportion of reads retained. The abundances were square root transformed and Bray–Curtis dissimilarity indices between samples were calculated in PRIMER 6 (PRIMER-E, Lutton, UK). The Chao 1 statistic was calculated in QIIME to estimate the total number of OTUs in each size fraction of each sample, and, therefore, the degree of undersequencing. Although this statistic can be sensitive to sequencing error because of its use of singleton OTU counts, this is unlikely to have a large effect as OTUs were clustered at the 0.97 sequence identity threshold. Environmental measurements and generation of distance matrix Environmental data were collected from CTD casts at each sample site. Pressure, dissolved oxygen concentration and water temperature measurements were collected with CTD instruments. Salinity and concentrations of dissolved phosphate, nitrate and silicate were obtained from hydrochemical analysis of seawater samples collected in Niskin bottles during CTD casts [36] . These samples were collected at discrete depths, and the hydrochemical sample closest to the depth of the relevant biological sample was selected. The exceptions were samples 32 and 33 (49.5° S, 115° E), for which nitrate concentrations were not available, and sample 29 (53.2° S, 115° E) for which phosphate concentration was not available. In these cases, a reading from the appropriate depth was substituted from the nearest available cast (50.0° S, 115° E for samples 32 and 33; 53.8° S, 115° E for sample 29). Pressure values were QUOTE transformed to reduce right skew [37] , and the combined instrument and hydrochemical data were used to create environmental profiles for each sample. The variables were normalized and a Euclidean distance matrix was generated in PRIMER 6. distLM multivariate analysis [38] was performed to confirm the selection of physicochemical variables and explore their relationship with taxonomic composition. In PRIMER 6, all possible combinations of variables (‘BEST selection’) were explored by distLM, and the models (sets of variables) that best fit the taxonomic dissimilarity matrix (adjusted R 2 as the fitness measure) were selected. The relationship between the resulting model and the taxonomic dissimilarity between samples was visualized by dbRDA ordination. To generate a spatial distance matrix, pairwise ellipsoidal distances between samples (including difference in depth) were calculated using INVERS3D (National Oceanic and Atmospheric Administration, Silver Springs, USA). Generation of advection distance matrix Advection distances between the sites were computed using three-dimensional velocity data from a hydrodynamic numerical ocean model in combination with a Lagrangian trajectory toolset. The ocean model used was the Southern Ocean State Estimate (SOSE) [39] , a numerical model of the SO based on the Estimating the Circulation and Climate of the Ocean machinery [40] and constrained by a large set of in situ and remote-sensed observations. SOSE has been validated in the SO [41] , [42] . Here the 5-day averaged three-dimensional velocity fields for the period January 2005–December 2007 were used on a 1/6° horizontal resolution and with 42 vertical levels. The Connectivity Modeling System [43] v1.1 was used to integrate virtual Lagrangian particles within the SOSE velocity fields. For each site, 100 particles were released every 5 days (with a total of 22,000 particles per site). The particles were released at the latitude and depth of the site, evenly spaced in a 1° zonal line centred at the site longitudes. The particles were then advected for 100 years, looping through the 3 years of available velocity fields as described in ref. 44 . Three-dimensional locations of the particles were saved every 5 days. The trajectory of each particle was analysed to detect encounters between particles and sample sites. An encounter was defined as the vector between any two consecutive 5-day particle locations intersecting a box bounded by ±0.2° of latitude, ±0.5° of longitude and ±50 m of depth from a sample site. Only the first encounter between any particle and sample was counted. Four pairs of samples (10/11, 12/13, 16/17 and 21/22), where a DCM sample was taken directly below a surface sample within the mixed layer, were too close to act as separate particle release sites. For these samples, simulated particle releases were performed for only one of the pair, and the generated encounters were attributed to both. For all samples pairwise, the mean time in seconds between a particle being released from one sample and encountering the other was calculated. Pairwise advective distance between samples was defined as the mean of these two directional mean times between each sample in the pair. This metric was selected to ensure advective flows, which may be of high biological relevance, such as a small number of particles quickly transported between sites were appropriately weighted when paired with flows of lower biological relevance, such as a large number of particles transported between sites over decades. To ensure the results were robust to this choice of metric, subsequent statistical tests were repeated with pairwise advective distance redefined as the mean time for all pairwise encounters. The pairwise distance between the surface/DCM samples discussed above was set to zero. For pairs of samples that did not yield mutual encounters (47 pairs, all including at least one AABW sample; see Results), the distance was set to the maximum run time of the simulation (100 years). To ensure these constraints were not unduly influencing the results, subsequent statistical tests were rerun without the surface/DCM samples, for which particle releases were not simulated, and AABW samples (see ‘Testing of advection effect’ below). Ordination of distances and comparison to water masses Ordinations of the taxonomic, environmental and advection distance matrices were produced by nMDS using custom R scripts. Analysis of similarities (ANOSIM) was performed in PRIMER 6 to test for statistically significant differences between water masses in each of these three factors. Right-tailed P -values for each ANOSIM test were computed using 999 random label permutations of one of the test matrices. Testing of advection effect Mantel tests were performed in Pattern Analysis, Spatial Statistics and Geographic Exegesis version 2 (ref. 45 ). To test for and quantify distance and environment effects, partial Mantel tests were performed comparing the taxonomic matrix with the spatial then the environmental matrices, with the remaining matrix held constant. To test the hypothesis that advection shapes SO microbial assemblages independent of distance and environment effects, a partial Mantel test was performed comparing the taxonomic and advection matrices, with both the spatial and environmental matrices held constant. Right-tailed P -values for all tests were calculated using 999 random label permutations of one of the test matrices. To ensure that the result was not unduly influenced by the samples to which the 100-year ceiling was applied (all AABW; see Results) and those for which particle releases were not simulated (samples 11, 13, 17 and 22), the test was repeated with these samples removed. To confirm that the advection effect was directional, that is, ‘upstream’ sites were acting as sources of diversity to ‘downstream’ sites, SourceTracker [46] was used to identify sources of OTUs in each sample. Each sample was sequentially designated a sink, with the remaining samples as potential sources, and the most probable proportion of OTUs originating from each potential source determined over 100 randomised trials per sample. Spearman’s rank correlation was then calculated between the SourceTracker-predicted source proportions and particle encounter source proportions for each sample pairwise, with right-tailed P -value determined by permutation. To explore the role of taxonomic resolution in detecting a significant advection effect, OTU clustering was repeated as above at sequence similarity thresholds of 0.80, 0.85, 0.90, 0.95, 0.99 and 1.00. Generation of relative abundance profiles and partial Mantel tests were performed as above. Accession codes: Pyrosequencing reads for this project have been deposited in the Sequence Read Archive (under Project Accession PRJNA194155, Sample Accessions SAMN01991086 – SAMN01991160 . How to cite this article: Wilkins, D. et al. Advection shapes Southern Ocean microbial assemblages independent of distance and environment effects. Nat. Commun. 4:2457 doi: 10.1038/ncomms3457 (2013).